Non-equilibrium dynamics of an unstable quantum pendulum explored in a spin-1 Bose–Einstein condensate A pendulum prepared perfectly inverted and motionless is a prototype of unstable equilibrium and corresponds to an unstable hyperbolic fixed point in the dynamical phase space. Here, we measure the non-equilibrium dynamics of a spin-1 Bose–Einstein condensate initialized as a minimum uncertainty spin-nematic state to a hyperbolic fixed point of the phase space. Quantum fluctuations lead to non-linear spin evolution along a separatrix and non-Gaussian probability distributions that are measured to be in good agreement with exact quantum calculations up to 0.25 s. At longer times, atomic loss due to the finite lifetime of the condensate leads to larger spin oscillation amplitudes, as orbits depart from the separatrix. This demonstrates how decoherence of a many-body system can result in apparent coherent behaviour. This experiment provides new avenues for studying macroscopic spin systems in the quantum limit and for investigations of important topics in non-equilibrium quantum dynamics. The inverted pendulum represents a hyperbolic fixed point, which is an unstable equilibrium in the classical limit. Phase orbits passing close to these points have exponentially diverging periods, and the orbits passing exactly through these points form a separatrix between librational and rotational motion of the pendulum with an infinite period. If the pendulum is prepared perfectly in this orientation, the classical equations of motion predict that it will not evolve. In reality, if perfect preparation was possible, thermal fluctuations of the pendulum would still perturb the pendulum from the metastable orientation and lead to oscillation. Even at zero temperature, unavoidable quantum fluctuations would lead to evolution [1] , [2] . Although mechanical pendulums operating at the quantum limit are currently unavailable in the lab, it is possible to study quantum many-body systems that have similar dynamical behaviour [3] , [4] , [5] . The equilibrium states, domain formation and spin dynamics of spinor condensates have been studied in many experiments [6] , [7] , [8] , [9] , [10] , [11] , [12] , [13] , [14] , [15] , [16] , [17] . In particular, observation of coherent spin oscillations have confirmed the mean-field pendulum model for small condensates [4] , [9] , [10] . Spin evolution has been previously observed from metastable spin states in many experiments [6] , [8] , [13] , [14] , [15] , [16] , [17] , however, the experiments have not yet demonstrated spin dynamic in agreement with quantum calculations, except in the perturbative, low-depletion limit at very short times (where a Bogoliubov expansion around the mean field can be used) [12] , [13] , [17] , or for conditions where the mean-field approach suffices. Here, we are able to observe quantum spin dynamics that agree well with quantum calculations and demonstrate a rich array of non-Gaussian fluctuations. The experiment uses spin-1 atomic Bose condensates [6] , [18] , [19] with ferromagnetic interactions tightly confined in optical traps such that spin domain formation is energetically suppressed. In this case, the non-trivial dynamical evolution of the system occurs only in the internal spin variables, and the mean-field dynamics of the system can be described by a non-rigid pendulum similar to the two-site Bose–Hubbard model [20] , [21] . The system is fully integrable in both the quantum [22] and classical [21] , [23] limits, and provides the opportunity to explore non-equilibrium quantum dynamics that are not captured by mean-field approaches, and can be solved exactly with Schrödinger’s equation. The condensate is prepared in a state corresponding to a hyperbolic fixed point in the spin-nematic phase space. Although this state is non-evolving in the mean-field limit, the quantum solution yields intricate spin-mixing dynamics exhibiting non-linear quantum revivals for zero magnetic field [22] and a quantum carpet of highly non-Gaussian fluctuations [24] . At finite fields, the dynamics are similar [25] , [26] , although they occur on a timescale favourable for experimental observation. In both cases, the evolution occurs along a separatrix of the phase space and is driven by quantum fluctuations that are absent from the mean-field theory solutions [23] , [26] . Spin population evolution The experiment begins with a rubidium-87 condensate, initialized in the f =1, m f =0 hyperfine ground state and held in a high magnetic field. The condensate is rapidly quenched through a quantum phase transition by lowering the field [27] , [28] , whereby the initial state is now a highly non-equilibrium but metastable state of the final Hamilitonian. The condensate is then allowed to freely evolve and the spin populations are measured for different evolution times. The experiment is repeated many times so as to acquire sufficient statistics to determine the full probability distributions of the populations. The main results of the paper are shown in Fig. 1 (top), which shows the measured probability density of the relative population of the m f =0 state, ρ 0 , versus evolution time. 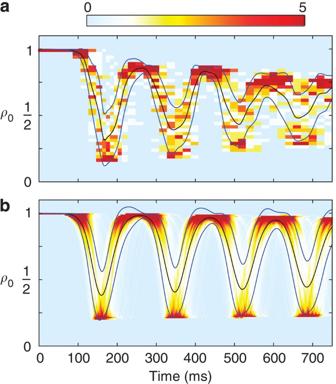Figure 1: Time evolution of spin populations. Probability density of the fractional population of the condensate in themf=0 state,ρ0, as a function of time. The curves show the mean,(black line) and±σ(blue lines). (a) Experimental data showing the results of 50 runs at each evolution time placed into 40 bins. The mean andσcurves have been smoothed using a cubic spline. (b) Quantum calculation using the initial atom number, magnetic field ramp and atom loss rate measured in the experiment. The Fock state probabilities |cp|2, placed into 100 bins, are plotted. Figure 1: Time evolution of spin populations. Probability density of the fractional population of the condensate in the m f =0 state, ρ 0 , as a function of time. The curves show the mean, (black line) and± σ (blue lines). ( a ) Experimental data showing the results of 50 runs at each evolution time placed into 40 bins. The mean and σ curves have been smoothed using a cubic spline. ( b ) Quantum calculation using the initial atom number, magnetic field ramp and atom loss rate measured in the experiment. The Fock state probabilities | c p | 2 , placed into 100 bins, are plotted. Full size image The experimental results are compared with a quantum calculation using the spin interaction Hamiltonian [22] , [24] , [25] , [26] , [29] : in the Fock basis, | N 1 , N 0 , N −1 〉, where N i are the number of atoms in the three spin-1 Zeeman states. Here, are the bosonic annihilation operators and are the corresponding number operators. λ (<0 for ferromagnetic interactions) and q ( B 2 ) characterize the inter-spin and Zeeman energies, respectively. The spin-dependent binary collisions restrict the dynamical evolution to states that conserve both the total number of atoms N i =Σ i N i and the projection of angular momentum along the quantization axis M = N 1 − N −1 . Starting from the initial state |0, N , 0〉, consisting of all N atoms in the m f =0 state, the evolution is constrained to final states of the form Σ p c p | p, N −2 p, p 〉. Hence, the solution to the quantum many-body problem is fully enumerated by the time dependence of the Fock state amplitudes, c p ( t ). To compare the measurements to the theory, we note that the measured probability density of ρ 0 = N 0 / N is effectively a determination of the probabilities | c p | 2 , averaged over the experimental detection resolution. The experimental results are in good overall agreement with the quantum calculation, particularly for early times. Both the experiment and theory exhibit a long pause (80 ms) before any population evolution is apparent. After this pause, the spin population executes a regular damped oscillation. Non-gaussian distributions of spin populations It is clear that the mean and standard deviation ( σ ) are insufficient to fully characterize the distribution of ρ 0 for both the experiment and theory, since for much of the evolution the mean does not pass through the highest probability density, indicating a significant skew in the distribution. This point is reinforced in Fig. 2b , which shows the full probability distributions for several evolution times, along with the theoretical predictions. The highly non-Gaussian nature of the distributions are a direct manifestation of the quantum spin dynamics. To characterize the non-Gaussian distribution, we determine several cumulants (linearly independent alternatives to the central moments), κ n from the data. The mean, σ and the third to sixth cumulants are shown in Fig. 3 compared with the quantum simulation. Overall, the measured cumulants are in good agreement with the predicted cumulants from the simulation. The population revival in the second oscillation predicted from the simulation is clearly seen in the mean, σ and third cumulant, but is less obvious in higher cumulants. 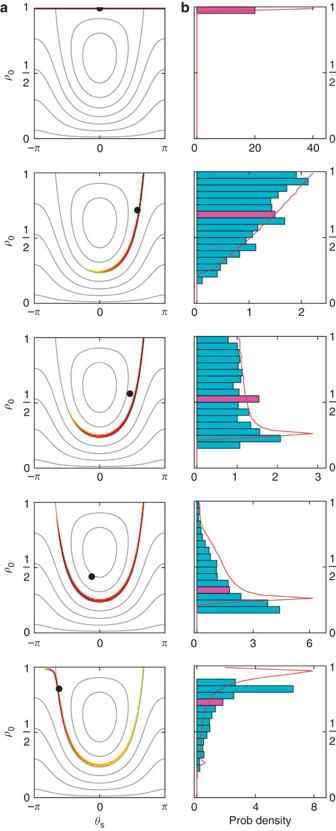Figure 2: Full probability distributions ofρ0. Evolution on the semi-classical phase space (left column) and histograms of the measured spin population,ρ0(right) for different evolution times after the quench, 15, 130, 140, 170 and 240 ms. (a) The simulations use the semi-classical equations of motion together with a quasi-probability distribution for the initial state. The mean value forρ0andθsare indicated with a black dot. (b) The histogram bars for each evolution time depict the measured probability density ofρ0for over 900 experimental runs, and the red line represents the simulation. The purple bar in each histogram represents the bin in which the mean ofρ0is located. Figure 2: Full probability distributions of ρ 0 . Evolution on the semi-classical phase space (left column) and histograms of the measured spin population, ρ 0 (right) for different evolution times after the quench, 15, 130, 140, 170 and 240 ms. ( a ) The simulations use the semi-classical equations of motion together with a quasi-probability distribution for the initial state. The mean value for ρ 0 and θ s are indicated with a black dot. ( b ) The histogram bars for each evolution time depict the measured probability density of ρ 0 for over 900 experimental runs, and the red line represents the simulation. The purple bar in each histogram represents the bin in which the mean of ρ 0 is located. 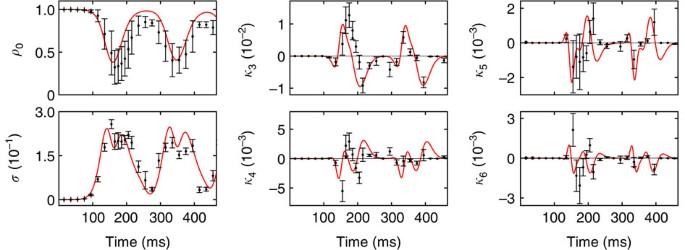Figure 3: Evolution ofρ0cumulants. The mean value ofρ0,σ, and the third through sixth cumulants,κn,n=3–6. The odd cumulants are on top, and the even cumulants are on the bottom. In each plot, the black markers represent the results of 50 experimental runs, and the error bars are estimated using a bootstrap method for the third cumulant and higher. The red curves are the prediction of the quantum simulation including loss. Full size image Figure 3: Evolution of ρ 0 cumulants. The mean value of ρ 0 , σ , and the third through sixth cumulants, κ n , n =3–6. The odd cumulants are on top, and the even cumulants are on the bottom. In each plot, the black markers represent the results of 50 experimental runs, and the error bars are estimated using a bootstrap method for the third cumulant and higher. The red curves are the prediction of the quantum simulation including loss. Full size image To understand the origin of the non-Gaussian fluctuations, it is helpful to consider the semi-classical limit of the spin Hamiltonian. Mean-field states of a spin-1 condensate can be written as ψ =(ζ +1 , ζ 0 , ζ −1 ) T where and ρ i =|ζ i | 2 = N i / N are the fractional spin populations. The conservation of magnetization m =( N 1 − N −1 )/ N constrains the populations ρ ±1 =(1− ρ 0 ± m )/2, and for the m =0 case that is relevant for these experiments, the spin dynamics are determined by the mean field equivalent to equation 1 [21] . Here, x =2 ρ 0 −1 and θ s = θ +1 + θ −1 −2 θ 0 are canonically conjugate variables and c =2 Nλ is the spinor dynamical rate. This Hamiltonian has the form of a classical non-rigid pendulum and is similar to the double-well Bose–Hubbard model that has been used to study Josephson effects in condensates [3] , [5] . The Hamiltonian can also be written using a phase space of the spin vector S i and nematic (quadrupole) tensor Q ij matrix operators for the spin-1 system: (ref. 17 ). The phase spaces for both of these forms are shown in Fig. 4 , where it is clear that the ρ 0 , θ s phase space corresponds to a projection of the spin-nematic phase space. 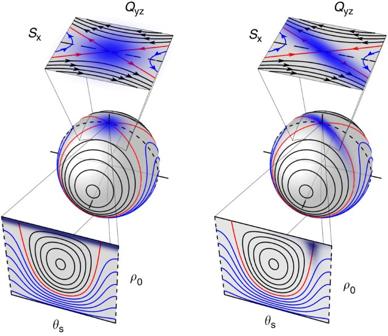Figure 4: Phase space. The evolution of the spin state following the quench is depicted on two relevant phase spaces of the spin-1 system: the {ρ0,θs} phase space (lower left), and the {Sx,Qyz,Qzz} spin-nematic Bloch sphere (centre). The left illustration represents the initial state, while the right illustration shows the system after a finite amount of evolution. The distributions for both cases have been exaggerated for illustrative purposes. A zoom-in of the hyperbolic fixed point at the pole is shown (top) with arrows indicating the orbit directions. Theρ0,θsphase space represents a Mercator projection of one of the degenerate hemispheres. Figure 4: Phase space. The evolution of the spin state following the quench is depicted on two relevant phase spaces of the spin-1 system: the { ρ 0 , θ s } phase space (lower left), and the { S x , Q yz , Q zz } spin-nematic Bloch sphere (centre). The left illustration represents the initial state, while the right illustration shows the system after a finite amount of evolution. The distributions for both cases have been exaggerated for illustrative purposes. A zoom-in of the hyperbolic fixed point at the pole is shown (top) with arrows indicating the orbit directions. The ρ 0 , θ s phase space represents a Mercator projection of one of the degenerate hemispheres. Full size image The initial state of the system following the quench is indicated in the different phase spaces in Fig. 4 using quasi-probability distributions of the initial state determined from the quantum uncertainties [17] . On the spin-nematic sphere, the state corresponds to a minimum uncertainty state centred at the pole. The pole is a hyperbolic fixed point lying at the intersection of the separatrix that separates the librational and rotational orbits of the system. In the ρ 0 , θ s phase space, the distribution in ρ 0 is tightly packed at the top of the phase space with random spinor phase. In the absence of quantum fluctuations, the state initialized exactly on the hyperbolic fixed point is non-evolving. However, quantum fluctuations populate a family of orbits that straddle the fixed point, and subsequent evolution leads to phase flow along the unstable manifolds of the separatrix. In the short term, this creates squeezed states with negligible change in ρ 0 (ref. 17 ). As evolution proceeds, the phase, θ s , converges towards the separatrix separating the librational and rotational trajectories, and the population starts to evolve along it. The separatrix has a divergent period [21] , and so the states disperse significantly due to the different evolution rates of nearby energy contours. It is this dispersion, together with the shape of the orbit, that gives rise to the highly non-Gaussian probability distributions. For longer times, the system evolves along the separatrix, which forms a closed homoclinic orbit in the spin-nematic space. Population evolution from the metastable state is exponentially sensitive to initial population in the m f =±1 states [13] . At the earliest evolution time studied (15 ms), the total population in these states is measured to be <30 atoms, which represents an upper bound limited by atom detection noise [17] . Initial populations at this level affect the duration of the initial pause and first oscillation minimum, but not the overall character of the evolution [24] . According to simulation, our results are consistent with no pollution ( Supplementary Fig. S1 and Supplementary Discussion , Effect of initial state impurities). For evolution times beyond >250 ms, it is necessary to include the effects of atomic loss in the theory. The lifetime of the condensate τ =1.8 s is only a factor of 10 larger than the spin evolution timescale ( ∼ 150 ms), hence one expects that loss has an important role in the long-term dynamics. We explore this question in Fig. 5 , where we compare quantum calculations without loss, quantum calculations including uncorrelated loss and the experimental data. Uncorrelated atom loss is incorporated into the calculation using quantum Monte Carlo techniques. The loss causes the overall magnetization M to execute a random walk with a restoring tendency towards M =0. 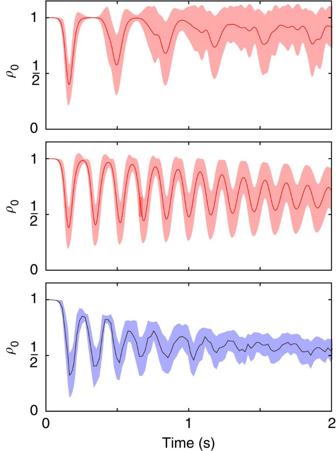Figure 5: Long-term evolution ofρ0. The top graph shows the quantum calculation without loss. The middle graphs shows the calculation including the effects of uncorrelated atom loss. The bottom graph shows the measured data. In each plot, the mean value is shown as a solid line, and the shaded envelopes correspond toσ. Figure 5: Long-term evolution of ρ 0 . The top graph shows the quantum calculation without loss. The middle graphs shows the calculation including the effects of uncorrelated atom loss. The bottom graph shows the measured data. In each plot, the mean value is shown as a solid line, and the shaded envelopes correspond to σ . Full size image For the first 250 ms of evolution corresponding to the first spin oscillation, the effects of loss are not discernible between the two calculations, and the experimental data are in good agreement with both. Beyond 250 ms, there are significant differences between the two quantum calculations. The spin population of the calculation without loss nearly returns to the initial value and then experiences a long pause followed by complex multi-frequency oscillations. The calculation with loss however exhibits steady oscillations with one dominant frequency and a slowly decreasing amplitude centred on the ground state populations. In the semi-classical picture, the apparent damping of the calculation without loss derives from the dispersion about the separatrix in Fig. 2 . The effect of loss is to eventually move the orbits away from the separatrix, which turns off this dispersion and leads to more regular oscillations. Although the inclusion of loss into the model makes a significant improvement in the agreement of long-term dynamics (>250 ms) with the experimental results, it is clear that this simple loss model is inadequate to fully replicate the measurements at longer time scales. Although the experimental data and the simulations with loss are qualitatively similar, there is clearly more dissipation in the experiment as the amplitude of the oscillations damp more quickly and the standard deviation decreases. In future work, we intend to further investigate the damping of the spin dynamics and its connection to thermalization of isolated quantum systems subject to loss. Similar investigations are ongoing using one-dimensional condensate systems [30] , [31] , [32] , [33] , and it will be interesting to explore the similarities and differences in these completely different systems. Finally, we believe that our results point the way to future explorations of quantum many-body spin systems, including thermalization and ergodicity crossing a quantum phase transition [34] , [35] , investigations of Hamiltonian monodromy [28] and other non-linear phenomena, finite temperature effects and dynamic stability. The combination of an exactly solvable Hamiltonian with a quantum phase transition together with demonstrated dynamics in the quantum regime should provide unique insights to these important topics. Experiment We prepare a condensate of N =38,500±500 87 Rb atoms in the | f =1, m f =0〉 hyperfine state in a high magnetic field (2 G). The condensate is tightly confined in an optical dipole trap with trap frequencies of 250 Hz. To initiate dynamical evolution, the condensate is quenched below the quantum critical point by lowering the magnetic field to a value 210 mG and then allowed to freely evolve for a set time. The trap is then turned off and a Stern–Gerlach field is applied to separate the m f components during 22 ms time-of-flight expansion. The atoms are probed for 400 μs with three pairs of orthogonal laser beams, and the resulting fluorescence signal is collected by a CCD camera with >90% quantum efficiency. Simulations The primary simulation method used to compare with the data is the numerical integration of the second quantized form of the Hamiltonian equation 1 ( Supplementary Methods , Second quantized calculations). Two different techniques were used to model the loss in the system. The first method involved decreasing the inter-spin energy, λ , with the number of atoms ( λ N −3/5 ) ( Supplementary Methods , Loss models: scaling the inter-spin energy). The second, more rigorous method involved the use of a quantum Monte Carlo techniques with the collapse operators ( Supplementary Methods , Loss models: quantum Monte Carlo). The mean-field phase space diagrams in Fig. 2 were created using a semi-classical simulation. Loss in this simulation was modelled similar to the first technique used in the quantum simulations, with the spinor dynamical rate, c =2 Nλ and λ N −3/5 ( Supplementary Methods , Mean-field calculations: semi-classical simulations). The quantum dynamics of the system were captured using an appropriate quasi-probability distribution obtained from the quantum noise of the initial Fock state ( Supplementary Fig. S2 and Supplementary Methods , Mean-field calculations: quasi-probability distributions). The simulations use a spinor energy, , chosen to match the population dynamics, and the other parameters ( B , N ) are chosen to match the experimental conditions. How to cite this article: Gerving, C.S. et al. Non-equilibrium dynamics of an unstable quantum pendulum explored in a spin-1 Bose–Einstein condensate. Nat. Commun. 3:1169 doi: 10.1038/ncomms2179 (2012).